A node-based switch for preferential distribution of manganese in rice Mineral nutrients, such as manganese, are required for the development of plants and their reproductive organs, but these can be toxic if accumulated at high concentrations. Therefore, plants must have a system for preferentially delivering an adequate amount of minerals to these organs for active growth and development, while preventing mineral overaccumulation in the face of changing environments. Here we show that a member of the Nramp transporter family, OsNramp3, functions as a switch in response to environmental Mn changes. OsNramp3 is constitutively expressed in the node, a junction of vasculatures connecting leaves, stems and panicles. At low Mn concentration, OsNramp3 preferentially transports Mn to young leaves and panicles. However, at high Mn concentration, the OsNramp3 protein is rapidly degraded within a few hours, resulting in the distribution of Mn to old tissues. Our results reveal the OsNramp3-mediated strategy of rice for adapting to a wide change of Mn in the environment. Mineral nutrients required for a plant’s growth and development in soil vary widely from deficient to excess levels, and are dependent on many factors, including pH, moisture, redox potential and cation-exchange capacity of soil, microbial activity and fertilizer application [1] . Their availability to plants also fluctuates spatially and temporally. Therefore, plants must have a fine system to deal with environmental changes, acquiring an adequate amount of mineral to meet cellular requirements at low external concentration, while preventing harmful overaccumulation at high external concentration. Maintaining a balanced supply of mineral nutrients to different tissues could be achieved at different steps. The first step is the regulation of uptake by the roots. Some transporters, such as iron transporter (IRT1) and boron transporter (BOR1), have been shown to be regulated at the transcriptional level or/and post-translational level [2] , [3] , [4] . For example, the expression of IRT1 was upregulated under Fe-limited condition [2] . On the other hand, the BOR1 protein was rapidly degraded in response to high B supply [4] . However, some other transporters for mineral uptake are consistently expressed. For example, a major rice transporter (OsNramp5) for manganese (Mn) uptake does not respond to external low and high Mn concentrations [5] . Therefore, a different regulatory system for dealing with environmental changes is required. After uptake by the roots, mineral nutrients are delivered to different tissues in the above-ground parts of plants. In rice and other gramineous plants, the distribution control of minerals to different tissues occurs in nodes. A rice culm has 13–16 nodes, with only the upper 4 or 5 separated by long internodes. Each node has a similar structure, which is characterized by remarkably developed vascular systems composing of enlarged vascular bundles (EVBs) and regular/diffuse vascular bundles (RVB/DVBs) [6] , [7] . EVBs in a node have a huge xylem area and are connected with a vascular bundle in a leaf and a lower node. On the other hand, RVB/DVBs are originated at the node surrounding the EVB and are connected to the upper node or panicle [7] , [8] . Therefore, the node is an important place for delivering nutrients from the roots to the developing tissues or panicles through intervascular transfer, which transfers nutrients from the transpirational stream in the xylem of EVBs into the xylem or phloem of the RVB/DVBs [6] , [7] , [8] . This preferential distribution to the developing tissues and panicles are especially important for plant growth and development under limited nutrient conditions. On the other hand, under nutrient excess conditions, this preferential distribution should be switched off to avoid growth damage due to overaccumulation. Previous physiological studies have shown that plants are able to change the distribution pattern in response to environmental changes. For example, the Mn distribution pattern in barley changes with Mn supply conditions [9] . Under Mn-sufficient condition, Mn taken up by the roots was distributed to expanded leaves. Under Mn-deficient condition, Mn was rapidly accumulated at the shoot basal region and then preferentially distributed to the youngest leaf [9] , [10] . However, molecular mechanisms underlying different distribution patterns in response to environmental changes are poorly understood. Mn is an essential metal for plant growth and development, which is involved in many biological processes, such as water-splitting activity in photosystem II, elimination of superoxide and various secondary metabolisms. The uptake of Mn in the roots is mediated by OsNramp5, a member of the natural resistance-associated macrophage proteins (Nramp) family transporter in rice [5] . The expression of OsNramp5 does not respond to external Mn supply levels, and Mn uptake and accumulation in the shoots increases with increasing external Mn concentrations ranging from submicromolar to hundreds of micromolars levels without affecting the growth [5] , [11] . This raises the question of how rice delivers the necessary amount of Mn to the developing tissues under Mn-limiting condition, while preventing Mn overaccumulation in the face of wide changes in external Mn concentrations. In the present study, we found that a node-localized Mn transporter, OsNramp3, functions as a switch for regulating Mn distribution in rice for dealing with variable changes of Mn in the environment. Under Mn-limited conditions, OsNramp3 preferentially transports Mn to the developing young leaf, crown root tips and panicle. However, under Mn-excess condition, OsNramp3 protein is rapidly degraded, resulting in altered distribution of Mn to the older leaves following transpiration. OsNramp3 was highly expressed in rice node As Mn distribution in rice may be regulated in the node, we examined the expression profile of Nramp family genes in rice node I at the flowering stage, because some of the Nramp proteins have been reported to transport Mn [5] . In the rice genome, there are seven members belonging to the Nramp family [5] , but only OsNramp3 showed a high expression in the node I ( Fig. 1a ). OsNramp3 (Os06g0676000 in RAP-DB (Rice Annotation Project Database) [12] ; http://rapdb.dna.affrc.go.jp/ ) encodes a putative membrane protein with 550 amino acids containing 11 predicted transmembrane domains (by SOSUI [13] ; http://bp.nuap.nagoya-u.ac.jp/sosui/ ). OsNramp3 shows identity of 45.2%, 46.2%, 59.6% and 60.0%, with OsNramp1, OsNramp5, AtNramp1 and AtNramp6, respectively, at the amino acid level ( Supplementary Fig. S1 ). 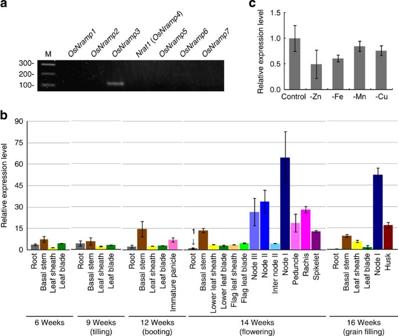Figure 1: Expression pattern ofOsNramp3. (a)The expression of seven riceNrampgenes in the node I at the flowering stage. The expression was investigated by RT–PCR with 26 cycles followed by agarose gel electrophoresis. (b) Relative expression ofOsNramp3in various tissues at different growth stages. Rice was grown in a paddy field until ripening and various tissues were sampled. (c) Response ofOsNramp3expression to metal deficiency in basal stem. Rice was cultivated in a nutrient solution with (control) or without Zn, Fe, Mn, or Cu for 1 week. The expression level was determined by quantitative real-time RT–PCR. Expression relative to the root at flowering stage (b) and to control condition (c) is shown.HistoneH3andActinwere used as internal standards. Data are means ±s.d. of three biological replicates. Difference was not significant inc(P>0.05 by Tukey’s test). Figure 1: Expression pattern of OsNramp3 . ( a )The expression of seven rice Nramp genes in the node I at the flowering stage. The expression was investigated by RT–PCR with 26 cycles followed by agarose gel electrophoresis. ( b ) Relative expression of OsNramp3 in various tissues at different growth stages. Rice was grown in a paddy field until ripening and various tissues were sampled. ( c ) Response of OsNramp3 expression to metal deficiency in basal stem. Rice was cultivated in a nutrient solution with (control) or without Zn, Fe, Mn, or Cu for 1 week. The expression level was determined by quantitative real-time RT–PCR. Expression relative to the root at flowering stage ( b ) and to control condition ( c ) is shown. HistoneH3 and Actin were used as internal standards. Data are means ±s.d. of three biological replicates. Difference was not significant in c ( P >0.05 by Tukey’s test). Full size image Expression pattern and response to metal deficiency We further investigated the expression pattern of OsNramp3 in different organs at various growth stages of rice grown in a paddy field. OsNramp3 showed a higher expression in the nodes (node I–III and basal stem containing unelongated nodes) throughout the growth period ( Fig. 1b ), although the expression was also detected in other organs at a low level. The highest expression was observed in the uppermost node I at the flowering and grain-filling stage. The expression of OsNramp3 was unaffected by deficiency of essential metals, including Zn, Fe, Mn and Cu ( Fig. 1c ). Subcellular localization of OsNramp3 To investigate the subcellular localization of the OsNramp3 protein, a fusion gene of OsNramp3 and GFP was transiently introduced into onion epidermal cells by particle bombardment ( Supplementary Fig. S2 ). Green fluorescence of the fusion protein was localized at the plasma membrane. By contrast, green fluorescence protein (GFP) alone was localized in the cytosol and the nucleus. OsNramp3 expression in yeast To examine which metal OsNramp3 transports, we expressed it in yeast for transport assays. In a yeast mutant Δ smf1 defective in Mn uptake, the expression of OsNramp3 rescued the growth under Mn-limited condition induced by Mn-chelator EGTA ( Fig. 2a ). On the other hand, OsNramp3 was not able to complement the Fe uptake in the yeast mutant Δ fet3fet4 under Fe-limited condition induced by Fe(II)-chelator BPDS (4,7-biphenyl-1,10-phenanthroline-disulphonic acid; Fig. 2b ). Growth inhibition by Cd was also not altered by the OsNramp3 expression ( Fig. 2c ). These results indicate that OsNramp3 functions as an influx transporter for Mn but not for Fe and Cd in yeast. 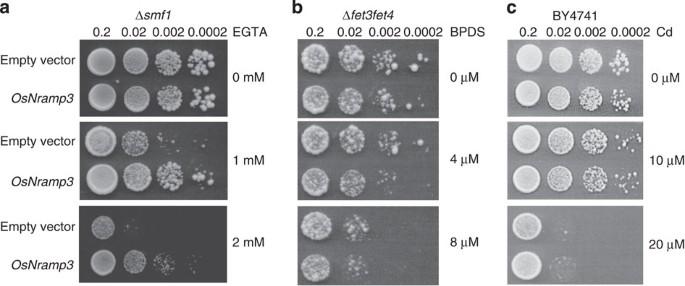Figure 2: Metal transport activity assay of OsNramp3 in yeast. OsNramp3or empty vector was introduced into yeast mutant strain Δsmf1defective in Mn uptake (a) or Δfet3fet4defective in Fe uptake (b), or WT strain BY4741 (c). The yeast was cultured on the plate with or without Mn-chelator EGTA (a), Fe(II)-chelator BPDS (b) or Cd (c) at 30 °C for 3 (a,c) or 5 (b) days. Figure 2: Metal transport activity assay of OsNramp3 in yeast. OsNramp3 or empty vector was introduced into yeast mutant strain Δ smf1 defective in Mn uptake ( a ) or Δ fet3fet4 defective in Fe uptake ( b ), or WT strain BY4741 ( c ). The yeast was cultured on the plate with or without Mn-chelator EGTA ( a ), Fe(II)-chelator BPDS ( b ) or Cd ( c ) at 30 °C for 3 ( a , c ) or 5 ( b ) days. Full size image Phenotypic analysis of OsNramp3 knockout and knockdown lines To investigate the role of OsNramp3 in rice, we obtained a T-DNA insertion mutant at the 12th exon of the gene (3A-01364 in RISD; http://www.postech.ac.kr/life/pfg/risd/ ). The expression of OsNramp3 at the 3′-untranslated region was not detected in the T-DNA insertion line, indicating that this mutant ( nramp3 ) is a knockout line (Supplementary Fig. S3a). In addition, we prepared knockdown lines by RNA interference (RNAi). The expression of OsNramp3 in the shoot basal region was reduced by 2/3 to 1/4 in five independent RNAi lines compared with that in the wild type (WT; Supplementary Fig. S3b ). The sequence of the OsNramp3 open reading frame (ORF) in two corresponding WTs, WT1 (cv. Dongjin) for T-DNA insertion line and WT2 (cv. Nipponbare) for RNAi lines is identical. When the WT rice (cv. Dongjin) and the knockout mutant were grown hydroponically under Mn-sufficient conditions at the vegetative growth stage, there were no visible differences in growth between the two lines ( Fig. 3a ). However, when grown under Mn-deficient condition, chlorosis in the new leaf, a growth defect and necrosis in the developing crown root tips of nramp3 was observed ( Fig. 3a,b and Supplementary Fig. S4 ). The RNAi lines also showed chlorosis in the new leaf and necrosis in the developing crown roots under Mn-deficient condition ( Supplementary Fig. S4 ). The SPAD value (indicator of chlorophyll content) of the newest leaf was decreased in the knockout line and four of five knockdown lines at 0.05 μM low Mn supply ( Supplementary Fig. S4b ). One RNAi line (line 9) did not show different SPAD value from the WT rice, because the expression suppression of this line was very weak ( Supplementary Fig. S3b ). The growth of the roots and young leaf (leaf 6) was also significantly decreased in the four knockdown lines under Mn-deficient condition ( Supplementary Fig. S4c,d ). These results consistently indicate that the growth defect is caused by loss or suppression of OsNramp3 function. 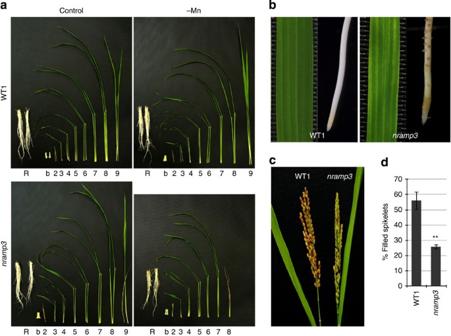Figure 3: Phenotype ofOsNramp3knockout line at different growth stage. (a) Growth at different Mn concentration. Three-week-old seedlings of WT rice (WT1, cv. Donjing) andOsNramp3knockout line (nramp3) were grown in a nutrient solution containing 0.5 μM Mn (control) or 0 (−Mn) for 12 days. Roots (R), shoot basal regions (b) and individual leaf (2–9 from older to younger) of two plants each are shown. (b) Phenotype of the youngest expanded leaf blade and crown root tip of plants without Mn supply for 12 days. (c) Phenotype of panicles. WT1 andnramp3were cultivated on soil until ripening. (d) Filled spikelet rate of WT1 andnramp3. Data are means±s.d. of four biological replicates. Significant difference at **P<0.01 by Tukey’s test. Figure 3: Phenotype of OsNramp3 knockout line at different growth stage. ( a ) Growth at different Mn concentration. Three-week-old seedlings of WT rice (WT1, cv. Donjing) and OsNramp3 knockout line ( nramp3 ) were grown in a nutrient solution containing 0.5 μM Mn (control) or 0 (−Mn) for 12 days. Roots (R), shoot basal regions (b) and individual leaf (2–9 from older to younger) of two plants each are shown. ( b ) Phenotype of the youngest expanded leaf blade and crown root tip of plants without Mn supply for 12 days. ( c ) Phenotype of panicles. WT1 and nramp3 were cultivated on soil until ripening. ( d ) Filled spikelet rate of WT1 and nramp3 . Data are means±s.d. of four biological replicates. Significant difference at ** P <0.01 by Tukey’s test. Full size image At the reproductive stage, knockout of OsNramp3 resulted in a decreased grain yield under paddy soil culture condition ( Fig. 3c ). Among yield components, only the filled spikelet rate was greatly reduced in the knockout line compared with the WT rice ( Fig. 3d , Supplementary Fig. S5 ). Metal analysis in different organs Metal analysis at the vegetative growth stage showed that there was no large difference in the Mn concentration in both the roots and shoots between WT rice and knockout or knockdown lines under both Mn-sufficient and -deficient conditions ( Fig. 4a,b ), indicating that loss or suppression of function of OsNramp3 did not significantly affect both the root uptake and root to shoot translocation of Mn. However, the concentration of Mn in the newest leaf (leaf 6) of the knockout and knockdown lines were only half of the WT rice under Mn-deficient condition ( Fig. 3c,d and Supplementary Figs. S6 ). The decrease of other metals, including Fe, Zn and Cu, was not observed in the knockout line ( Supplementary Fig. S7 ). The concentration of Mn, but not other metals, was also significantly decreased in the crown root tips of both knockout and knockdown lines ( Supplementary Fig. S8 ). At the reproductive stage, knockout of OsNramp3 resulted in a decrease in Mn concentration in the panicles, although the concentrations of Fe, Zn and Cu were not changed ( Fig. 4e and Supplementary Fig. S9 ). These results suggest that the high expression of OsNramp3 in the nodes is involved in preferential distribution of Mn to developing tissues, including the root tips, new leaves and panicles. 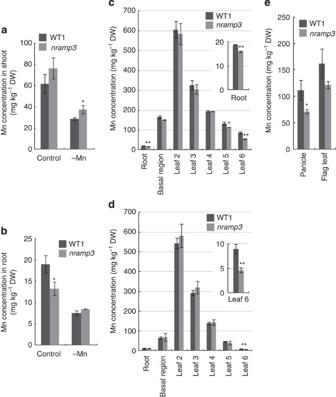Figure 4: Concentration of Mn in different organs. (a,b) Mn concentration in the shoots (a) and roots (b). Three-week-old seedlings of two WT rice and knockout line (nramp3) were grown in a nutrient solution containing 0.5 μM Mn (control) or 0 (−Mn) for 12 days. (c,d) Distribution of Mn in different organs. WT1 andnramp3seedlings were grown hydroponically till the six-leaf stage (3-week-old) and then subjected to 0.5 μM Mn (c) or 0 μM (d) for 1 week. (e) Mn concentration in immature panicles and flag leaf at the heading stage. Both WT1 andnramp3were grown in nutrient solution containing 0.5 μM Mn. Data are means ±s.d. of three biological replicates. Significant difference from WT1 at *P<0.05 and **P<0.01 by Student’st-test. Figure 4: Concentration of Mn in different organs. ( a , b ) Mn concentration in the shoots ( a ) and roots ( b ). Three-week-old seedlings of two WT rice and knockout line ( nramp3 ) were grown in a nutrient solution containing 0.5 μM Mn (control) or 0 (−Mn) for 12 days. ( c , d ) Distribution of Mn in different organs. WT1 and nramp3 seedlings were grown hydroponically till the six-leaf stage (3-week-old) and then subjected to 0.5 μM Mn ( c ) or 0 μM ( d ) for 1 week. ( e ) Mn concentration in immature panicles and flag leaf at the heading stage. Both WT1 and nramp3 were grown in nutrient solution containing 0.5 μM Mn. Data are means ±s.d. of three biological replicates. Significant difference from WT1 at * P <0.05 and ** P <0.01 by Student’s t -test. Full size image Labelling experiment with 54 Mn radioisotope To investigate the above suggestion, we performed a short-term labelling experiment with the 54 Mn radioisotope. Seedlings at the eight- to nine-leaf stage were pretreated with 0.05 and 50 μM Mn for 1 week and were fed with 54 Mn from the roots for 3 h. The eighth leaf was not expanded in rice pretreated with 0.05 μM Mn, whereas it was fully expanded in rice pretreated with 50 μM Mn. At low Mn supply (0.05 μM), 84% of Mn newly taken up was retained at the shoot basal region and 12% was delivered to the developing young leaf (unexpanded leaf 8) in the WT rice ( Fig. 5a ). The distribution to the older leaves was very low ( Fig. 5a ). By contrast, in the mutant, <60% of total Mn was retained in the basal region and the distribution to the developing leaf (leaf 8) was negligible ( Fig. 5a ). Most Mn was delivered to the older leaves following a transpiration-dependent distribution pattern ( Fig. 5a ). Interestingly, at high Mn concentration (50 μM), the Mn distribution in both the WT rice and the knockout line followed the transpiration rate, and the difference in the distribution pattern disappeared between two lines ( Fig. 5b ). Similar results were also observed in RNAi lines ( Supplementary Fig. S10 ). These results indicate that the OsNramp3-mediated distribution of Mn changes in response to external Mn concentrations. 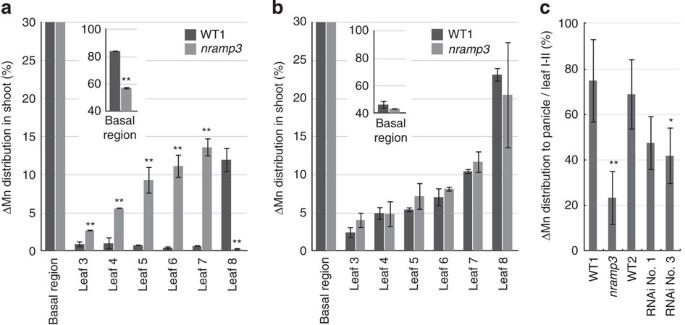Figure 5: Distribution of Mn in different organs. (a,b) Short-term distribution analysis of Mn at the vegetative stage. Seedlings (eight-leaf stage) pretreated with 0.05 (a) or 50 μM (b) Mn for 1 week were exposed to a nutrient solution containing54Mn for 3 h. (c) Short-term distribution analysis of54Mn at the heading stage. Each line grown hydroponically with 0.5 μM cold Mn till the heading was used.54Mn-labelled 0.5 μM Mn was fed from the roots for 24 h. Distribution ratio of Mn newly taken up in panicle/(leaf I+II) was calculated. Data are means ±s.d. of three (a,b) or four (c) biological replicates. Significant difference from the corresponding wild types at *P<0.05 and **P<0.01 by Tukey’s test. Figure 5: Distribution of Mn in different organs. ( a , b ) Short-term distribution analysis of Mn at the vegetative stage. Seedlings (eight-leaf stage) pretreated with 0.05 ( a ) or 50 μM ( b ) Mn for 1 week were exposed to a nutrient solution containing 54 Mn for 3 h. ( c ) Short-term distribution analysis of 54 Mn at the heading stage. Each line grown hydroponically with 0.5 μM cold Mn till the heading was used. 54 Mn-labelled 0.5 μM Mn was fed from the roots for 24 h. Distribution ratio of Mn newly taken up in panicle/(leaf I+II) was calculated. Data are means ±s.d. of three ( a , b ) or four ( c ) biological replicates. Significant difference from the corresponding wild types at * P <0.05 and ** P <0.01 by Tukey’s test. Full size image At the heading stage, the distribution ratio of labelled 54 Mn to the panicles was much lower in the nramp3 mutant and RNAi lines compared with that in the corresponding WT rice ( Fig. 5c ). Tissue localization of OsNramp3 protein We investigated tissue-specificity of the localization of OsNramp3 protein by immunohistochemical staining using an antibody against the carboxy terminus region of OsNramp3. In the root and leaf of rice treated without Mn for 1 week, OsNramp3 protein was only detected in the phloem parenchyma cells of the vascular tissues ( Fig. 6a–c ). At the basal node, OsNramp3 protein was localized at the xylem and phloem regions, in particular the vascular bundles ( Fig. 6d,e ). No signals were detected in the nramp3 knockout line ( Fig. 6f ). In RNAi lines, much weaker signals of OsNramp3 protein was detected ( Supplementary Fig. S11 ). In addition, staining without the primary antibody also yielded no signal ( Supplementary Fig. S11d ), indicating the high specificity of the antibody. 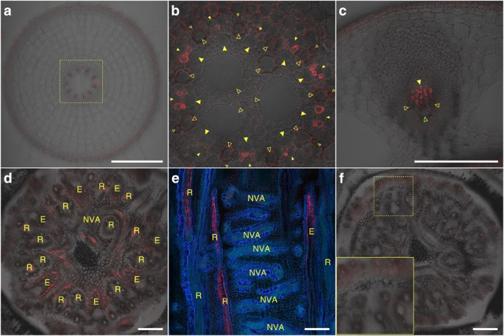Figure 6: Localization of OsNramp3 protein at the vegetative stage. Five-week-old seedlings of WT1 andnramp3grown hydroponically with 1/2 Kimura B solution were used for immunostaining of OsNramp3 (red colour). (a) Cross-section of a crown root of WT1. (b) Magnified image of yellow dotted box ina. (c) Cross-section of a leaf sheath of WT1. Cross (d) and longitudinal (e) section of a basal node of WT1. (f) Cross-section of a basal node ofnramp3. Open arrowheads inbandcindicate xylem vessels. Closed arrowheads inbandcindicate sieve tube and phloem region, respectively. RVB in node (R), EVB in node (E) and nodal vascular anastomosis (NVA) are shown indande. Blue colour ineshowed cell wall ultraviolet autofluorescence. Inset infshowed background red fluorescence from thick cell wall in the magnified image of yellow dotted box. Scale bars, 200 μm. Figure 6: Localization of OsNramp3 protein at the vegetative stage. Five-week-old seedlings of WT1 and nramp3 grown hydroponically with 1/2 Kimura B solution were used for immunostaining of OsNramp3 (red colour). ( a ) Cross-section of a crown root of WT1. ( b ) Magnified image of yellow dotted box in a . ( c ) Cross-section of a leaf sheath of WT1. Cross ( d ) and longitudinal ( e ) section of a basal node of WT1. ( f ) Cross-section of a basal node of nramp3 . Open arrowheads in b and c indicate xylem vessels. Closed arrowheads in b and c indicate sieve tube and phloem region, respectively. RVB in node (R), EVB in node (E) and nodal vascular anastomosis (NVA) are shown in d and e . Blue colour in e showed cell wall ultraviolet autofluorescence. Inset in f showed background red fluorescence from thick cell wall in the magnified image of yellow dotted box. Scale bars, 200 μm. Full size image As OsNramp3 is highly expressed in the nodes ( Fig. 1 ), we further examined OsNramp3 localization at three different levels of the basal stem, which contain several unelongated basal nodes ( Fig. 7 ). In the lower basal node, which is armed with fully developed old leaf and crown roots, OsNramp3 protein was only detected at the xylem parenchyma cells surrounding EVBs, which include xylem transfer cells (XTCs) ( Fig. 7a,b ). At the middle basal node, which bears expanded source leaf and developing crown roots, OsNramp3 signal in the xylem parenchyma around the EVBs were relatively weaker than that in the lower nodes ( Fig. 7c,d ), but additional signals were detected in the phloem region of the RVBs ( Fig. 7c,d ). In the upper basal node connecting with developing young leaf but no developing crown roots, OsNramp3 was also detected in both the xylem parenchyma cells of the EVBs and the phloem parenchyma cells of the RVBs ( Fig. 7e,f ), although signals in the EVBs were much weaker than that of the middle basal nodes. These distinct localizations together with the Mn distribution in different leaves ( Fig. 4c,d ) indicate that OsNramp3 has a different role in the different position of the basal stem. In the lower basal node, OsNramp3 mediates the uptake of Mn from the transpiration stream in xylem vessels of EVBs connected to the older leaves into surrounding xylem parenchyma cells, whereas in the upper basal node it is responsible for reloading Mn into the phloem of RVBs connected to the developing young leaves. 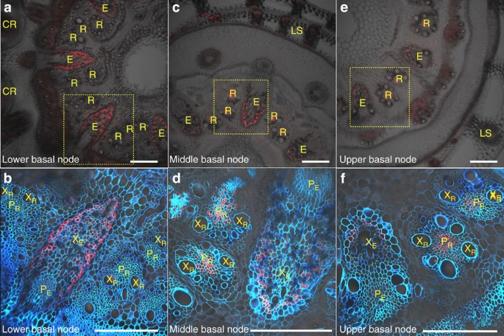Figure 7: Immunostaining of OsNramp3 protein at different levels of basal stem. Four-week-old seedlings of WT2 grown hydroponically with 1/2 Kimura B solution were treated with −Mn nutrient solution for 4 days and the basal stem used for immunostaining of OsNramp3 (red colour). (a,b) Cross-section at the lower part of basal stem. (c,d) Cross-section at the middle part of basal stem. (e,f) Cross-section at the upper part of basal stem. (b,d,f) showed magnified image of yellow dotted box ina,cande, respectively. Blue colour inb,dandfshowed cell wall autofluorescence. Crown root (CR), leaf sheath (LS), RVB in node (R), EVB in node (E), xylem and phloem region of R and E (XR, PR, XE, PE) are shown. Scale bars, 200 μm. Figure 7: Immunostaining of OsNramp3 protein at different levels of basal stem. Four-week-old seedlings of WT2 grown hydroponically with 1/2 Kimura B solution were treated with −Mn nutrient solution for 4 days and the basal stem used for immunostaining of OsNramp3 (red colour). ( a , b ) Cross-section at the lower part of basal stem. ( c , d ) Cross-section at the middle part of basal stem. ( e , f ) Cross-section at the upper part of basal stem. ( b , d , f ) showed magnified image of yellow dotted box in a , c and e , respectively. Blue colour in b , d and f showed cell wall autofluorescence. Crown root (CR), leaf sheath (LS), RVB in node (R), EVB in node (E), xylem and phloem region of R and E (X R , P R , X E , P E ) are shown. Scale bars, 200 μm. Full size image Rapid degradation of OsNramp3 protein in response to high Mn We investigated the response of OsNramp3 to different Mn concentrations at the transcript and protein level. The expression level of OsNramp3 in different organs was not changed by Mn concentrations ranging from 0 to 50 μM at the vegetative growth stage ( Supplementary Fig. S12a ). A short exposure (2 h) to high Mn levels also did not change the expression ( Supplementary Fig. S12a ). The expression level of OsNramp3 in node I was also not affected by Mn concentrations at the reproductive stage ( Supplementary Fig. S12b ). However, immunostaining showed that the protein level was rapidly changed in response to high Mn. In the xylem parenchyma cells of EVB at the middle part of basal node, OsNramp3 was observed at the peripheral area of the cells in rice grown in Mn-free solution for 4 days ( Fig. 8a ). However, the localization of OsNramp3 changed from the cell surface to a vesicle-like organelle as early as 0.5 h after the plants were exposed to 50 μM Mn ( Fig. 8b ). This internalization of OsNramp3 protein progressed up to 4 h ( Fig. 8c–e ) and finally the signals disappeared at 24 h after the exposure ( Fig. 8f ). In the phloem parenchyma cells of RVB, similar internalization and degradation of OsNramp3 were observed ( Supplementary Fig. S13 ), although the progression was slightly slower than that in the xylem parenchyma cells ( Supplementary Fig. S13 and Fig. 8 ). 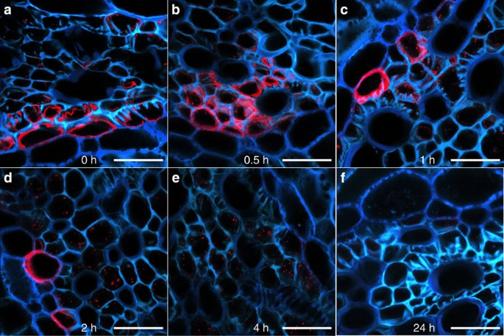Figure 8: Rapid response of OsNramp3 protein localization to excess Mn in basal node xylem parenchyma cell. Four-week-old seedlings of WT2 grown hydroponically with 1/2 Kimura B solution were pretreated with −Mn nutrient solution for 4 days and then were transferred to nutrient solution containing 50 μM Mn. After 0 (a), 0.5 (b), 1 (c), 2 (d), 4 (e) and 24 h (f), basal stems were sampled for immunostaining of OsNramp3 (red colour). Projection image was constructed fromZ-stack images at xylem of EVBs in the middle part of the basal stem. Blue colour showed cell wall autofluorescence. Scale bars, 20 μm. Figure 8: Rapid response of OsNramp3 protein localization to excess Mn in basal node xylem parenchyma cell. Four-week-old seedlings of WT2 grown hydroponically with 1/2 Kimura B solution were pretreated with −Mn nutrient solution for 4 days and then were transferred to nutrient solution containing 50 μM Mn. After 0 ( a ), 0.5 ( b ), 1 ( c ), 2 ( d ), 4 ( e ) and 24 h ( f ), basal stems were sampled for immunostaining of OsNramp3 (red colour). Projection image was constructed from Z -stack images at xylem of EVBs in the middle part of the basal stem. Blue colour showed cell wall autofluorescence. Scale bars, 20 μm. Full size image We further investigated the change of OsNramp3 protein when the plants pretreated with high Mn were transferred to a Mn-free solution. At 2 h after the transfer, the signal of OsNramp3 was recovered first in the vesicles ( Supplementary Fig. S14 ). With the progression of time, the signal gradually became stronger and finally moved to the plasma membrane at 96 h. All these results indicate that OsNramp3 protein in the node changes in response to different Mn concentrations. Compared with internalization and degradation caused by Mn excess, the relocalization process caused by Mn deficiency was slower. Localization of OsNramp3 in node I As OsNramp3 showed the highest expression in the node I at the reproductive growth stage ( Fig. 1b ), we also investigated its localization and response to Mn concentrations with immunostaining. At the flowering stage, OsNramp3 protein was mainly observed at the XTCs and other xylem parenchyma cells surrounding the EVB of node I ( Fig. 9a,b ), which are similar to the localization in the unelongated vegetative nodes ( Figs 6 and 7 ). Signals at the phloem region of DVBs were also detected but were weaker than that in the xylem parenchyma cells of EVBs ( Fig. 9a ). When excess Mn was supplied (1,000 μM Mn for 4 days), OsNramp3 protein was internalized to a vesicle-like organelle and the signal mostly disappeared ( Fig. 9c,d ). However, the expression level of OsNramp3 transcript in node I was unaffected by high Mn concentration ( Supplementary Fig. S12b ). 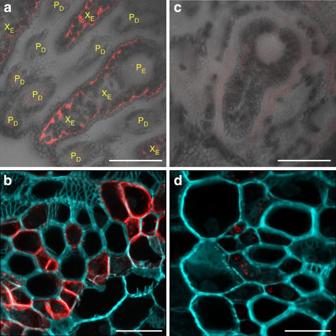Figure 9: Immunostaining of OsNramp3 protein at the reproductive stage. WT2 plants were grown hydroponically with 0.5 μM Mn throughout the growth (a,b) or 1,000 μM Mn for last 4 days (c,d). Node I at the flowering stage was used for immunostaining of OsNramp3 (red colour). (a,c) Cross-section of node I. (b,d) Magnified image of xylem area of EVB. Blue colour inbanddshowed cell wall autofluorescence. Xylem and phloem region of EVBs (XE, PE) and phloem region of DVBs (PD) are shown. Scale bars, 200 μm (a,c) and 20 μm (b,d). Figure 9: Immunostaining of OsNramp3 protein at the reproductive stage. WT2 plants were grown hydroponically with 0.5 μM Mn throughout the growth ( a , b ) or 1,000 μM Mn for last 4 days ( c , d ). Node I at the flowering stage was used for immunostaining of OsNramp3 (red colour). ( a , c ) Cross-section of node I. ( b , d ) Magnified image of xylem area of EVB. Blue colour in b and d showed cell wall autofluorescence. Xylem and phloem region of EVBs (X E , P E ) and phloem region of DVBs (P D ) are shown. Scale bars, 200 μm ( a , c ) and 20 μm ( b , d ). Full size image Preliminary investigation of internalization mechanism To investigate the pathway involved in the internalization and degradation of OsNramp3 protein, we conducted a double staining with the endocytotic dye, FM4-64, and the OsNramp3 antibody. When the internalization was induced by 50 μM Mn for 2 h in the basal nodes, small vesicles containing OsNramp3 protein were mostly colocalized with FM4-64-labelled endosomes ( Supplementary Fig. S15 ). These results suggest that the rapid internalization of OsNramp3 protein caused by high Mn is controlled by endocytotic process, although further work is required. Rice is able to grow under both upland and paddy field, where Mn concentration in the soil solution varies from submicromolar to hundreds of micromolars. We found that OsNramp3 has a crucial role in dealing with such wide ranges of Mn concentrations in the environment at both the vegetative and reproductive growth stage. The uptake of Mn in rice roots is mediated by OsNramp5 (ref. 5 ). However, Mn uptake increases with increasing external Mn concentrations and there is no regulation of OsNramp5 expression in response to Mn supply level [5] . After the uptake, Mn is translocated to the shoot, together with water flow driven by the transpiration, and is subsequently distributed to different organs. If the distribution of Mn follows the transpiration, more Mn will be allocated to the older organs, such as mature leaves, because they have larger surface area and, therefore, higher transpiration. On the other hand, the developing leaves and crown roots have small surface area and low transpiration, but require high Mn for active cell division and elongation. Therefore, a preferential distribution to these new organs and tissues is required, especially under limited Mn condition. At the vegetative growth stage, OsNramp3 protein is localized at the XTCs of EVBs and the phloem region of RVBs in basal nodes under limited Mn condition ( Figs 6 and 7 ). Our results show that OsNramp3 has two roles in Mn distribution in the basal nodes. One is that OsNramp3 at the XTCs functions in the uptake of Mn from the transpiration stream in the xylem vessels of EVB ( Fig. 10a ). XTCs are characterized by increased cell surface area due to cell wall ingrowth [14] , making efficient uptake possible. The other is that OsNramp3 at the phloem region of RVB functions in reloading Mn to the phloem ( Fig. 10 ). RVB is connected to developing leaves and crown roots, which require relatively high Mn for growth. Therefore, OsNramp3 is required for the preferential distribution of Mn to the developing organs at the vegetative growth stage. This is supported by the phenotype of the knockout or knockdown lines. Knockout or knockdown of OsNramp3 resulted in decreased Mn in the youngest leaf and crown root tips ( Fig. 4 , and Supplementary Figs S6 and S8 ), causing leaf chlorosis and root necrosis ( Fig. 3 and Supplementary Fig. S4 ). 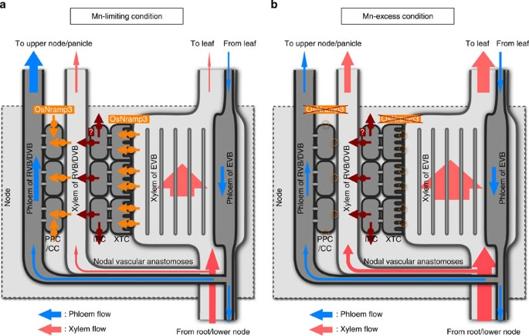Figure 10: Schematic presentation ofOsNramp3role in Mn distribution. (a) Role ofOsNramp3under Mn-limited condition. Mn in decelerated transpiration flow is unload by OsNramp3 at the XTC of EVB, and then released to apoplast between EVB and RVB/DVB by another unidentified transporter, followed by reloading Mn to the phloem of RVB/DVB by OsNramp3 expressed in adjacent phloem parenchyma cells (PPC) and companion cells (CC). (b) Role ofOsNramp3under Mn-excess condition. OsNramp3 protein is rapidly internalized and degraded in response to excess Mn via post-translational process(es). Therefore, Mn distribution to each organ follows transpiration rate through the xylem. Figure 10: Schematic presentation of OsNramp3 role in Mn distribution. ( a ) Role of OsNramp3 under Mn-limited condition. Mn in decelerated transpiration flow is unload by OsNramp3 at the XTC of EVB, and then released to apoplast between EVB and RVB/DVB by another unidentified transporter, followed by reloading Mn to the phloem of RVB/DVB by OsNramp3 expressed in adjacent phloem parenchyma cells (PPC) and companion cells (CC). ( b ) Role of OsNramp3 under Mn-excess condition. OsNramp3 protein is rapidly internalized and degraded in response to excess Mn via post-translational process(es). Therefore, Mn distribution to each organ follows transpiration rate through the xylem. Full size image When the plants are exposed to high Mn concentration, the expression of OsNramp3 transcript was unaffected ( Supplementary Fig. S12 ), but OsNramp3 protein was rapidly internalized and degraded ( Fig. 8 and Supplementary Fig. S13 ), indicating that OsNramp3 is regulated at the post-translational level but not at the transcriptional level in response to external Mn changes. Degradation of OsNramp3 results in an alternation of Mn distribution in different organs; more Mn is distributed to the leaves with high transpiration ( Fig. 10b ). Therefore, the distribution pattern of Mn becomes similar between WT rice and knockout/knockdown lines ( Fig. 5 and Supplementary Fig. S10 ). This rapid degradation of OsNramp3 could avoid Mn toxicity in the developing tissues due to its overaccumulation. In old leaves, Mn will be detoxified and OsYSL6 is involved in this process by transporting Mn–NA complex from apoplast to symplast [11] . Interestingly, post-translational control of the Nramp transporter was also found in yeast. Yeast Smf1, a transporter for Mn uptake [15] , is also degraded in response to high Mn concentration. Trafficking from the plasma membrane to the vacuole occurs in yeast at high Mn [15] , but it remains to be investigated that whether similar mechanism for degradation of OsNramp3 is involved in rice. At the reproductive growth stage, upper nodes at the elongated stem are important for mineral distribution. In uppermost node I, which connects with the flag leaf and the panicle, OsNramp3 is mainly localized at the XTCs ( Fig. 9 ). Therefore, the role of OsNramp3 in node I is the same as that in basal node, that is, the uptake of Mn from the transpiration stream in the xylem vessels for preferential distribution to the panicle ( Fig. 10a ). Knockout of OsNramp3 resulted in a decrease in Mn concentration in the panicles, and subsequently low fertility ( Figs 3 and 4 ). OsNramp3 in node I also undergoes internalization and degradation similar to that in the basal node in response to high Mn ( Fig. 9 ). Recently, a few transporters involved in delivering minerals to the seeds have been reported, including Lsi6 for Si (ref. 16 ), OsLCT1 for Cd (ref. 17 ), OsYSL16 for Cu (ref. 18 ) and OsHMA2 for Zn and Cd (ref. 19 ). In Arabidopsis, AtNIP6;1, a boric acid channel is involved in preferential distribution of B at the nodal region [20] . However, it remains to be further examined whether these transporters respond to environmental changes like OsNramp3. In conclusion, OsNramp3 in the rice nodes functions as a switch for Mn distribution, which turns on or off the protein in response to fluctuating Mn concentrations. Under Mn-limited conditions, OsNramp3 localized in the nodes mediates intervascular transfer and preferential distribution of Mn to the developing tissues, including young leaves, crown root tips and panicles, to meet the Mn requirement for the growth ( Fig. 10a ). By contrast, under Mn-excess conditions, OsNramp3 is rapidly internalized and degraded to avoid toxicity of Mn due to overaccumulation in active developing tissues, and Mn is then delivered to the old leaves following transpiration-dependent manner ( Fig. 10b ). Post-translational regulation of OsNramp3 presents a strategy for rice to deal with variable Mn concentrations in the paddy soil environment. Plant materials and growth condition WT rice (WT1; cv. Dongjin, WT2; cv. Nipponbare), T-DNA insertion mutant lines (3A-01364) from RISD ( http://www.postech.ac.kr/life/pfg/risd/ ) and five independent RNAi lines described below were used. For hydroponic experiments, seeds were soaked in water overnight at 25 °C in the dark and then transferred to a net floating on 0.5 mM CaCl 2 solution. On day 7, seedlings were transferred to a 3.5-l plastic pot containing one-half-strength Kimura B solution [5] . The pH of this solution was adjusted to 5.6 and the nutrient solution was renewed every 2 days. For soil culture, three-week-old seedlings grown hydroponically were transplanted to a 3.5-l plastic pot filled with paddy soil. Tap water was supplied daily. Both hydroponic and soil culture plants were grown in a closed greenhouse at 25–30 °C under natural light. All experiments were repeated with at least three biological replicates. To compare the growth at different Mn concentrations, WT rice, knockout and knockdown lines (3-week-old) were exposed to a nutrient solution containing 0.05 and 0.5 μM Mn. After 1 week, the SPAD value of the youngest expanded leaf (leaf 5) was measured with a SPAD-5 chlorophyll metre (Konika Minolta, Japan). The roots, basal region and individual leaf were separately collected and their fresh weight was recorded. Cloning of full-length complementary DNA of OsNramp3 To isolate the full-length ORF sequence of OsNramp3 from the WT1 and WT2, total RNA was extracted from the basal stem region by using a RNeasy Plant Mini Kit (Qiagen) and were then converted to cDNA using the protocol supplied by the manufacturers of SuperScript II (Invitrogen). The full-length ORF was amplified by PCR using primers; 5′-AGATGAGCGGCCCAATGCAAC-3′ and 5′-CTAATCGAGATCAGAAGCAGTTC-3′, which were designed based on gene annotations in the RAP-DB ( http://rapdb.dna.affrc.go.jp/ ), Os06g0676000. Sequence comparison of OsNramp3 showed that there was no difference between WT1 and WT2. Alignment of amino acid sequences Peptide sequence alignment was generated by ClustalW using default setting ( http://clustalw.ddbj.nig.ac.jp/ ). Transmembrane domains were predicted with SOSUI ver. 1.11 ( http://bp.nuap.nagoya-u.ac.jp/sosui/ ). Preparation of OsNramp3 knockdown line To generate the RNAi knockdown line of OsNramp3 , we amplified a 383-bp fragment of OsNramp3 cDNA by PCR using a pair of primers (5′-AAAAAGCAGGCTGGAGGGCGATTCGACGG-3′ and 5′-AGAAAGCTGGGTGTCACAGGATCACAGTTAG-3′). We then cloned two copies of the fragment into the pANDA vector as inverted repeats according to Miki and Shimamoto [21] , and subsequently introduced the construct into rice (WT2, cv Nipponbare) using an Agrobacterium tumefaciens -mediated transformation system as described previously [22] . The expression level of the shoot basal region was determined in five RNAi lines randomly selected as described below. Expression analysis To investigate the expression pattern of OsNramp3 at different growth stages, 3-week-old seedlings of WT2 precultured hydroponically were transplanted to the paddy field of the Okayama University at mid June. Samples, including roots, basal stem, leaf sheath and leaf blade at the vegetative stage and roots, basal stem, lower leaf sheath, lower leaf blade, flag leaf sheath, flag leaf blade, immature panicle, node I–III, inter node II, peduncle, rachis spikelet and husk at the reproductive stages, were taken. For the metal-deficiency response analysis of OsNramp3 in the basal stem at the vegetative stage, 2-week-old seedlings (WT2) were exposed to a 1/2 Kimura B solution with or without Zn, Fe, Mn or Cu. After 1 week, the shoot basal region (1 cm above the roots) were sampled and subjected to RNA extraction. The metal-deficiency status has been confirmed by the expression induction of marker genes related to Fe-, Zn- or Cu deficiency [18] . For Mn response analysis, 2-week-old seedlings were exposed to a 1/2 Kimura B solution with 0, 0.05, 0.5, 5 or 50 μM Mn for 1 week. Rapid change from plants pretreated with 0 μM Mn for 1 week to 50 μM Mn for 2 h was also examined. The roots, shoot basal regions (0.5 cm above the roots) and shoots were sampled for RNA extraction. Total RNA was extracted by using an RNeasy Plant Mini Kit (Qiagen) followed by DNase I treatment, and then was converted to cDNA using the protocol supplied by the manufacturer of SuperScript II (Invitrogen). Specific cDNAs were amplified by Sso Fast EvaGreen Supermix (Bio-Rad) and quantitative real-time PCR was performed with the following primer sets for OsNramp3 ; 5′-CACACAAATTCAAAAGCCATTTCTG-3′ and 5′-CGATAGACCGTTGTGGAGAAGC-3′ on CFX384 (Bio-Rad). HistoneH3 and Actin were used as internal standards with primer pairs 5′-AGTTTGGTCGCTCTCGATTTCG-3′ and 5′-TCAACAAGTTGACCACGTCACG-3′ for HistoneH3 , and 5′-GACTCTGGTGATGGTGTCAGC-3′ and 5′-GGCTGGAAGAGGACCTCAGG-3′ for Actin . The relative expression was normalized based on these two genes by ΔΔCt method using the CFX Manager software (Bio-Rad). Subcellular localization of OsNramp3 The ORF of the OsNramp3 was amplified with PCR using primers (5′-TGTCGACATGAGCGGCCCAATGCAACG-3′ and 5′-TCCATGGAATCGAGATCAGAAGCAGTT-3′), and was inserted into CaMV 35S GFP vector. The resulting plasmid was designated OsNramp3-GFP . Gold particles with a diameter of 1 μm coated with OsNramp3-GFP or GFP alone were introduced into onion epidermal cells using particle bombardment (PDS-1000/He particle delivery system, Bio-Rad; http://www.bio-rad.com/ ) using 1,100 psi rupture disks. The cell wall was stained by propidium iodide. Plasmolysis was induced by 1 M mannitol. The GFP signal was observed with a confocal laser-scanning microscopy (LSM700, Carl Zeiss). OsNramp3 expression in yeast The cDNA fragment containing an entire ORF for OsNramp3 was amplified by RT–PCR using the primers 5′-AGGATCCAAGATGAGCGGCCCAATGCAAC-3′ and 5′-TCTCGAGCTAATCGAGATCAGAAGCAGTTC-3′. The fragment was directly cloned into the pYES2 vector (Invitrogen). After sequence confirmation, the resulting plasmid or the empty vector was introduced into yeast according to the manufacturer’s protocols (S.c. easy comp transformation kit, Invitrogen). The yeast strains used in this study were BY4741 ( MATa his2Δ0 met15Δ0 ura3Δ0 ), the Mn uptake-deficient mutant Δ smf1 ( MATa his2Δ0 met15Δ0 ura3Δ0 YOL122c::KanMX4 ) and the Fe uptake-deficient double-mutant DDY4 ( fet3fet4; MATa ade6 can1 his3 leu2 trp1 ura3 fet3-2::HIS3 fet4-LEU ). DDY4 was grown in media supplemented with 0.2 mM FeCl 3 . Complementation of the Δ smf1 phenotype was tested on a synthetic medium containing 2% galactose, 0.67% yeast nitrogen base without metals (BIO 101 Systems), 0.2% appropriate amino acids and 2% agar buffered at pH 6 with 50 mM Mes and supplemented with 0, 1 or 2 mM EGTA. Complementation of the DDY4 phenotype was tested on synthetic medium containing 2% galactose, 0.67% yeast nitrogen base without metals, 0.2% appropriate amino acids and 2% agar buffered at pH 5.5 with 50 mM Mes in the presence of 0, 4 or 8 μM BPDS. For evaluation of cadmium tolerance in yeast (BY4741), transformants were cultured and spotted on synthetic complete (SC)-uracil plates containing glucose or galactose, and were supplemented with 0, 10 or 20 μM CdSO 4 . After spotting at yeast-cell dilutions (optical densities at 600 nm of 0.2, 0.02, 0.002 and 0.0002), plates were incubated for 5 days at 30 °C. All yeast experiments were conducted at least three times independently and yielded same results. Immunohistological staining of OsNramp3 The synthetic peptide C-REDISSMQLPQQRTASDLD (positions 532–550 of OsNramp3) was used to immunize rabbits to obtain antibodies against OsNramp3. The obtained antiserum was purified through a peptide affinity column before use (1.0 mg protein per ml, 1/1,000 diluted for use). Basal nodes at the vegetative stage (4–5 weeks old seedlings) and node I at the flowering stage of WT1, WT2, nramp3 mutant and RNAi lines treated with various Mn concentrations were used for immunostaining of OsNramp3 protein as described previously [23] . For costaining with endocytotic dye, 50 μM FM4-64 were added to the nutrient solution containing 50 μM Mn and were supplied to rice from half-cut roots for 2 h. Fluorescence of secondary antibody (Alexa Fluor 555 goat anti-rabbit IgG, Molecular Probes) was observed with a confocal laser-scanning microscopy (LSM700; Carl Zeiss). Determination of metals in plant tissues The dried samples were digested with concentrated HNO 3 (60%) at a temperature up to 140 °C. The metal concentration in the digest solution was determined by atomic absorption spectrometry (Z-2000, Hitachi, Japan) and ICP-MS (7700X, Agilent Technologies) after dilution. Short-term distribution analysis of 54 Mn Seedlings of WT1, WT2, nramp3 and three independent RNAi lines were hydroponically grown to five-leaf stage (WT2 and RNAi lines) to six-leaf stage (WT1 and nramp3 ) and then subjected to a solution containing 0.05 or 50 μM cold Mn for 1 week. Before labelling experiment, leaf 1 and 2 were detached due to extremely small size. Two plants each were exposed to a 50-ml nutrient solution containing 54 Mn (80 kBq; 0.002 μM) in the presence of 0.05 or 50 μM cold Mn. After 3 h, individual leaf and shoot basal region (0–1 cm from the root–shoot junction) were sampled for radioactivity measurement. For analysis at the reproductive stage, WT1, WT2, nramp3 and two independent RNAi lines were grown hydroponically with 0.5 μM cold Mn till the heading and then were used for labelling experiment as described above. After 24 h, samples including each node, leaf and immature panicle were sampled. Radioactivity of each part was measured immediately by Auto Well Gamma System ARC-360 (Aloka). Distribution ratio of Mn newly taken up within the shoot was calculated based on the radioactivity of each part. Statistical analysis of data Statistics was performed by Student’s t -test or Tukey’s test. Significance was defined as * P <0.05 or ** P <0.01. How to cite this article: Yamaji, N. et al . A node-based switch for preferential distribution of manganese in rice. Nat. Commun. 4:2442 doi: 10.1038/ncomms3442 (2013). Accession codes: The nucleotide sequence data have been deposited in the DDBJ/EMBL/GenBank nucleotide sequence database under the accession code AB775807 .